Magnetically driven suppression of nematic order in an iron-based superconductor A theory of superconductivity in the iron-based materials requires an understanding of the phase diagram of the normal state. In these compounds, superconductivity emerges when stripe spin density wave (SDW) order is suppressed by doping, pressure or atomic disorder. This magnetic order is often pre-empted by nematic order, whose origin is yet to be resolved. One scenario is that nematic order is driven by orbital ordering of the iron 3 d electrons that triggers stripe SDW order. Another is that magnetic interactions produce a spin-nematic phase, which then induces orbital order. Here we report the observation by neutron powder diffraction of an additional fourfold-symmetric phase in Ba 1− x Na x Fe 2 As 2 close to the suppression of SDW order, which is consistent with the predictions of magnetically driven models of nematic order. There have been extensive investigations of the phase diagrams of the various iron arsenide and chalcogenide structures that display high temperature superconductivity with critical temperatures up to 55 K [1] , [2] , [3] , [4] . In common with other unconventional superconductors, such as the copper oxides, heavy fermions and organic charge-transfer salts, superconductivity is induced by suppressing a magnetically ordered phase, which generates a high density of magnetic fluctuations that could theoretically bind the Cooper pairs. Whether this is responsible for the high transition temperatures has not been conclusively established, but it makes the origin of the magnetic interactions an important issue to be resolved [5] , [6] . In nearly all the iron arsenides and chalcogenides, the iron atoms form a square planar net and the magnetic order consists of ferromagnetic stripes along one iron–iron bond direction that are antiferromagnetically aligned along the orthogonal iron–iron bond [6] , [7] . These systems are metallic and the Fermi surfaces, which are formed by the iron 3 d electrons, are nearly cylindrical with hole pockets at the centre of the Brillouin zone and electron pockets at the zone boundaries, all of similar size. In such an electronic structure, interactions between electrons near the two sets of pockets give rise to a spin density wave (SDW) order at the wave vector connecting them [8] . This itinerant picture is consistent with the wave vector of the observed antiferromagnetism, angle resolved photoemission (ARPES) measurements of the electronic structure [9] , [10] and the evolution of the dynamic magnetic susceptibility with carrier concentration [11] , [12] , [13] . However, any theory of the magnetic order also has to explain the structural transition that occurs at a temperature either just above or coincident with the SDW transition and lowers the symmetry from tetragonal ( C 4 ) to orthorhombic ( C 2 ). This is often referred to as nematic order, and the relation between nematicity, magnetic order and superconductivity has become one of the central questions in the iron-based superconductors [14] , [15] . At present, there are two scenarios for the development of nematic order and its relation to SDW order. In the first, the structural order is unrelated to magnetism and is driven by orbital ordering as the primary instability. The orbital ordering induces magnetic anisotropy and triggers the magnetic transition at a lower temperature by renormalizing the exchange constants [16] , [17] , [18] . This scenario is largely phenomenological, but there have been recent efforts to develop a microscopic basis [19] . In the second scenario, the structural order is driven by magnetic fluctuations, associated with the fact that striped SDW order can be along the x -axis (ordered momentum is Q X =(0, π)) or along the y -axis (ordered momentum is Q Y =(π, 0)). Theory predicts that the Z 2 symmetry between the X and Y directions can be broken above the true SDW ordering temperature that breaks O (3) spin symmetry, that is, the system distinguishes between Q X and Q Y without breaking time reversal symmetry [20] . The order parameter of this ‘Ising-spin-nematic state’ couples linearly to the lattice, inducing both structural and orbital order. The magnetic scenario has been developed for itinerant [8] , [20] and localized [21] , [22] , [23] , [24] electrons, and the phase diagrams are rather similar in the two approaches. Below we use the fact that the systems we study are metals and use an itinerant approach. Many of the observable properties are identical in both the orbital and magnetic scenarios, hindering a determination of the origin of nematicity. In the following, we report the discovery of a new magnetic phase in hole-doped Ba 1− x Na x Fe 2 As 2 (refs 25 , 26 ) at doping levels close to the suppression of magnetic order. This second phase, which occurs at temperatures below the conventional C 2 transition, restores C 4 rotational symmetry, indicating that the SDW order combines Q X and Q Y with equal weights. Such a second transition is highly unlikely in an orbital scenario because the breaking of symmetry of Q X and Q Y is a precondition for a magnetic transition to occur. However, it is known that such a phase is a possible solution of itinerant magnetic models for certain combinations of electronic interactions and/or Fermi surface geometries [8] , [27] , [28] , [29] . By going beyond our earlier Ginzburg-Landau analysis, we now show that the phase diagram is much richer than previously thought and that the C 4 phase becomes energetically favourable at higher doping levels, particularly in the range of phase coexistence with superconductivity [29] . We therefore view the observation of the transition to an SDW state, which does not break the symmetry between Q X and Q Y , as a strong indication that the nematic order is of magnetic origin. A magnetically driven C 4 phase also provides a natural explanation for the new phase observed in transport measurements in Ba 1− x K x Fe 2 As 2 under external pressure [30] and may explain anomalous diffraction results in Ba(Fe 1− x Mn x ) 2 As 2 (ref. 31 ), so it is probably present in other iron-based superconductors, although our calculations show that its stability is highly sensitive to details of the electronic structure. In the following, we describe the experimental evidence for a re-entrant C 4 phase in neutron and x-ray diffraction data on Ba 1− x Na x Fe 2 As 2 for x ≥0.24. We then summarize the results of theoretical calculations showing that such a phase is consistent with magnetically driven nematic order. Experiment We have conducted a detailed survey of the phase diagram of Ba 1− x Na x Fe 2 As 2 using neutron and x-ray powder diffraction [25] , following our recent investigation of the potassium-doped compounds [32] . In both the K-doped and Na-doped series, the addition of the alkali metal dopes holes into iron d -bands and reduces the transition temperature into the stripe phase from 139 K, in the parent compound BaFe 2 As 2 , to 0 at x ~0.25−0.3. One unusual feature of both series is that the antiferromagnetic and orthorhombic transitions are coincident and first-order over the entire phase diagram [33] , an observation that is quite unambiguous since both order parameters are determined from the same neutron powder diffraction measurement. Details of the synthesis and characterization of the polycrystalline samples and the powder diffraction measurements are given in the Methods section. We provide a comparison of the sample stoichiometries with earlier reports in Supplementary Note 1 . The only region of the sodium series where there are significant departures from the conventional behaviour observed in many iron-based superconductors is at 0.24≤ x ≤0.28 close to the suppression of the AF/O order. These compounds are all in the region where superconductivity coexists with magnetic order at low temperature. The results are summarized in Fig. 1 , where diffractograms are shown for three Bragg reflections at ( h , k , l )=(112), and , respectively, using tetragonal reciprocal lattice indices. The (112) reflection is a nuclear Bragg peak that splits when the symmetry is lowered to orthorhombic, while the other two reflections are magnetic Bragg peaks. 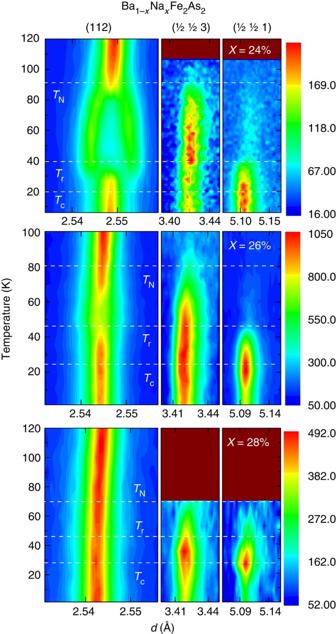Figure 1: Temperature dependence of powder neutron diffraction from Ba1−xNaxFe2As2. The first diffractogram is of HRPD data from the (112) Bragg peak (using tetragonal indices), which shows the orthorhombic transition atTNand the re-entrant tetragonal transition atTrinx=0.24 and 0.26. The symmetry is tetragonal at all temperatures inx=0.28. The other two diffractograms are of Wish data from magnetic Bragg peaks. Thedata show the onset of stripe SDW order atTN. Thedata show the onset of theC4SDW order atTr. The absolute intensities are arbitrary, but, to display all the plots on the same colour scale, theintensities have been multiplied by factors of 208, 200 and 144, and theby factors of 30, 20 and 60, forx=0.24, 0.26 and 0.28, respectively. The magnetic Bragg peaks show a significant reduction of intensity below the superconducting transition atTc, indicating the phase competition between magnetism and superconductivity. Figure 1: Temperature dependence of powder neutron diffraction from Ba 1− x Na x Fe 2 As 2 . The first diffractogram is of HRPD data from the (112) Bragg peak (using tetragonal indices), which shows the orthorhombic transition at T N and the re-entrant tetragonal transition at T r in x =0.24 and 0.26. The symmetry is tetragonal at all temperatures in x =0.28. The other two diffractograms are of Wish data from magnetic Bragg peaks. The data show the onset of stripe SDW order at T N . The data show the onset of the C 4 SDW order at T r . The absolute intensities are arbitrary, but, to display all the plots on the same colour scale, the intensities have been multiplied by factors of 208, 200 and 144, and the by factors of 30, 20 and 60, for x =0.24, 0.26 and 0.28, respectively. The magnetic Bragg peaks show a significant reduction of intensity below the superconducting transition at T c , indicating the phase competition between magnetism and superconductivity. Full size image At x =0.24 and 0.26, the transition into the C 2 ( Fmmm ) phase at T N ~70–90 K is clearly evident. However, at T r ~40–50 K, there is a second phase transition, not seen at x =0.22 (not shown), at which the orthorhombic splitting collapses and tetragonal C 4 ( I 4/ mmm ) symmetry is restored. The reflection, which shows the onset of stripe SDW order at T N , weakens in intensity in the C 4 phase, whereas the reflection strengthens considerably. This indicates that there is a strong spin reorientation with respect to the stripe SDW order when tetragonal symmetry is restored at T r . It was not possible to obtain an unambiguous refinement of the C 4 magnetic structure; hence, we cannot determine whether the reorientation is in-plane or out-of-plane. A full solution will require measurements on single crystals. At x =0.27 (not shown) and 0.28, the temperature variation of the and reflections show evidence of the same two magnetic transitions at T N and T r , although the orthorhombic splitting is too weak to be detected in the intermediate phase even on a high-resolution diffractometer like HRPD. These observations are summarized in the phase diagram of Fig. 2 , which shows that the new phase is confined to doping levels very close to the suppression of stripe SDW order. At x =0.24, the lower transition at T r is very sharp and appears to be first-order because there is evidence that up to 40% of the sample remains in the C 2 phase below T r . The C 2 phase fraction is reduced to 20% at x =0.26. It is not possible to determine whether there is phase coexistence at higher doping. Further details of the coexistence of C 2 and C 4 phases at x =0.24 and 0.26 are provided in Supplementary Note 2 . 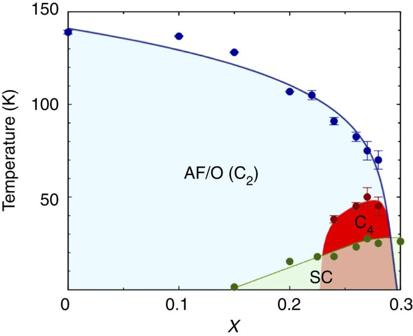Figure 2: Phase diagram of Ba1−xNaxFe2As2. The blue points are the coincident antiferromagnetic and orthorhombic transition temperatures,TN, into theC2phase, and the red points are the observed transition temperatures,Tr, into theC4phase, all measured by neutron diffraction. The green points are the superconducting transition temperatures,Tc, determined from magnetization data. The error bars represent the temperature interval in the neutron diffraction measurements. Figure 2: Phase diagram of Ba 1− x Na x Fe 2 As 2 . The blue points are the coincident antiferromagnetic and orthorhombic transition temperatures, T N , into the C 2 phase, and the red points are the observed transition temperatures, T r , into the C 4 phase, all measured by neutron diffraction. The green points are the superconducting transition temperatures, T c , determined from magnetization data. The error bars represent the temperature interval in the neutron diffraction measurements. Full size image Figure 1 shows that the C 4 phase competes with the superconductivity because there is a strong suppression of the magnetic peak intensities at temperatures below T c . This is similar to the phase competition between superconductivity and the C 2 phase seen in the electron-doped superconductors [34] , but much stronger than the phase competition observed in the Ba 1− x K x Fe 2 As 2 series [33] . Theory The itinerant description of magnetism in iron-based superconductors is built on the fact that the hole bands are centred around Q Γ =(0, 0) and the electron bands are centred at Q X =(π, 0) and Q Y =(0, π), respectively ( Fig. 3a ). The spin susceptibility is logarithmically enhanced at momenta connecting the hole and electron pockets, and SDW order develops even if the interaction is weak. The SDW order parameter is in general a combination of the two vector components Δ X and Δ Y with momenta (π, 0) and (0, π), respectively. For a model of perfect Fermi surface nesting (circular hole and electron pockets of equal radii) and only electron–hole interactions, SDW order determines | Δ X | 2 +| Δ Y | 2 but not the relative magnitudes and directions of Δ X and Δ Y . Away from perfect nesting, the ellipticity of the electron pockets and interactions between the electron bands break the degeneracy and lower the symmetry of the SDW order. Near T N , an analysis within a Ginzburg-Landau expansion in powers of Δ X and Δ Y shows that fourth-order terms select stripe magnetic order with either Δ X ≠0, Δ Y =0 or Δ Y ≠0, Δ X =0 (refs 8 , 20 ). Such an order simultaneously reduces the lattice C 4 symmetry down to C 2 . The order parameter in the stripe phase is shown schematically in Fig. 3b . 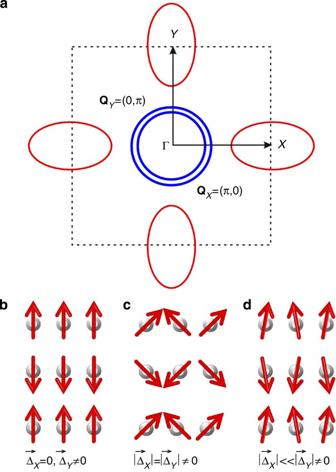Figure 3: Spin-nematic models of magnetic order. (a) The band-structure with two circular hole pockets at Γ and two electron pockets atXandY, using the unfolded Brillouin zone with one Fe atom per unit cell. The arrows refer to two equivalent nesting wave vectorsQX=(π, 0) andQY=(0, π). (b–d) Possible magnetic ground states of the Fe-lattice: (b) theC2antiferromagnetic stripe phase with ΔX=0 and ΔY≠0; (c) aC4magnetic state, in which |ΔX|=|ΔY|≠0, that is compatible with tetragonal lattice symmetry (this is one of several possible solutions of theC4magnetic structures); (d) magnetic order in which |ΔX| << |ΔY|≠0. Note that the Néel transition at low temperatures,Tr, from phase (b) to phase (c) is first order, while the transition from phase (b) to phase (d) is second order, in which an additional small component of ΔXappears belowTr. Our experiments are more compatible with scenario (c). Figure 3: Spin-nematic models of magnetic order. ( a ) The band-structure with two circular hole pockets at Γ and two electron pockets at X and Y , using the unfolded Brillouin zone with one Fe atom per unit cell. The arrows refer to two equivalent nesting wave vectors Q X =(π, 0) and Q Y =(0, π). ( b – d ) Possible magnetic ground states of the Fe-lattice: ( b ) the C 2 antiferromagnetic stripe phase with Δ X =0 and Δ Y ≠0; ( c ) a C 4 magnetic state, in which |Δ X |=|Δ Y |≠0, that is compatible with tetragonal lattice symmetry (this is one of several possible solutions of the C 4 magnetic structures); ( d ) magnetic order in which |Δ X | << |Δ Y |≠0. Note that the Néel transition at low temperatures, T r , from phase ( b ) to phase ( c ) is first order, while the transition from phase ( b ) to phase ( d ) is second order, in which an additional small component of Δ X appears below T r . Our experiments are more compatible with scenario ( c ). Full size image An issue that has not been discussed in detail until now is whether another magnetic ground state, in which both Δ X and Δ Y are non-zero, may appear at a lower temperature, as a result of non-linear effects. This might happen either via a first-order transition, in which case the most likely outcome is the state in which |Δ X |=|Δ Y | (see Fig. 3c ), or via a second-order transition, in which case the second order parameter appears continuously and likely remains relatively small down to T =0. To check for a potential second SDW transition, we needed to go beyond the previous Ginzburg-Landau analysis; hence, we solved non-linear coupled mean-field equations for Δ X and Δ Y over the entire temperature range and analysed which solution minimizes the free energy. This has revealed new features in the phase diagram not previously identified. In particular, we find that SDW order with Δ X = Δ Y , which breaks O (3) spin symmetry but preserves lattice C 4 symmetry, does emerge at low T , as the mismatch in hole and electron pocket sizes grows. We obtained this result by analysing the minimal three-band model with one hole and two electron pockets. For simplicity, we considered parabolic dispersions with where m i are band masses, ε 0 is the offset energy and μ is the chemical potential. The non-interacting Hamiltonian takes the form where i =1–3 label the bands, the summation over repeated spin indices α is assumed, and we shift the momenta of the fermions near the X and Y Fermi pockets by Q X and Q Y , respectively, writing . The interaction term in the Hamiltonian int contains all symmetry-allowed interactions between low-energy fermions, which include inter- and intra-band scattering processes [35] . We present the explicit form of int in the Supplementary Methods . The mean-field equations on Δ X and Δ Y are obtained by introducing and and using them to decouple four-fermion terms into anomalous quadratic terms with inter-band ‘hopping’, which depends on Δ X and Δ Y . We diagonalized the quadratic form, re-expressed c i , k α in terms of new operators and obtained a set of two coupled self-consistent equations for Δ X and Δ Y . We solved the mean-field equations numerically as a function of two parameters, δ 0 and δ 2 (see Supplementary Methods for details). The parameter δ 0 =2μ represents the mismatch in chemical potentials of the hole and electron pockets ( δ 0 =0 when the electron and hole pockets are identical). δ 2 = ε 0 m ( m x − m y )/(2 m x m y ) is proportional to the ellipticity of the electron pockets. We focused on the two SDW-ordered states, on the antiferromagnetic stripe state with Δ X ≠0 and Δ Y =0, in which C 4 -symmetry is reduced to C 2 , and the SDW state with Δ X = Δ Y , in which C 4 -symmetry is preserved. As we said, the two states are degenerate at zero ellipticity and perfect nesting, when δ 2 = δ 0 =0. Once the ellipticity becomes non-zero, the stripe state wins immediately below the Néel temperature T N . The C 4 -preserving state (with Δ X = Δ Y ) is a local maximum and is unstable at T ≤ T N . By solving the equations at lower temperature, we found that, at a finite δ 0 , the C 4 -preserving state also becomes locally stable below some T < T N , and, at an even lower T < T N , its free energy becomes smaller than that of the stripe phase, that is, at T = T r the system undergoes a first-order phase transition in which lattice C 4 symmetry gets restored (see Fig. 3c ). Because T N falls as the Fermi surface mismatch δ 0 increases, the new C 4 -preserving phase in practice exists only in a narrow region of the phase diagram close to the suppression of SDW order, as observed in Fig. 2 . We also analysed a four-pocket model with two hole pockets and found another scenario for a second SDW transition. Namely, the AF stripe order Δ Y initially involves only fermions from a hole pocket, which has higher density of states. Below some T < T N , fermions near the remaining hole pocket and near the electron pocket at X , not involved in the initial stripe order, also produce a SDW instability, and the system gradually develops the second order parameter | Δ X |, which distorts the stripe AF order. The corresponding low T -spin configuration is shown in Fig. 3d . In this case, however, the C 4 symmetry remains broken at all temperatures. Our experimental data taken as a function of doping are more consistent with a first-order transition and restoration of C 4 symmetry, although it is possible that the second scenario is realized under pressure [30] . We have demonstrated the existence of a wholly new magnetic phase that exists at the boundary between superconductivity and stripe magnetism, an observation that has important implications for the origin of magnetic and structural transitions in the iron-based superconductors. It is important to distinguish these new results from previous observations of a re-entrant tetragonal phase in electron-doped compounds, such as BaFe 2− x Co x As 2 (ref. 34 ). All those transitions were within the superconducting phase and have been shown to result from the competition between superconductivity and stripe SDW order [36] , [37] . The re-entrant phase that we report here occurs at temperatures that are more than twice as high as T c and so requires a different explanation. However, there is a similar competition between magnetism and superconductivity in the new phase evident from the partial suppression of the ordered magnetic moment below T c . We are unaware of any model of orbital order that would predict a re-entrant non-orbitally ordered phase at lower temperature. However, the prediction of spin-nematic models that a C 4 phase can become degenerate with the C 2 phase only at higher doping when the hole and electron Fermi surfaces are not as well-matched in size, and that the stability of the C 4 phase would be limited to a very narrow region close to the suppression of antiferromagnetism is borne out by the new data. Our results therefore provide strong evidence for the validity of an itinerant model of nematic order in the iron-based superconductors, in which the orbital reconstruction of the iron 3 d states is a consequence of magnetic interactions induced by Fermi surface nesting. Whether nematic order, or at least strong nematic fluctuations, is a prerequisite for superconductivity is another challenge to address in the future. Sample synthesis Mixtures of Ba, Na and FeAs were loaded in alumina tubes, sealed in niobium tubes under argon and sealed again in quartz tubes under vacuum. The mixtures were variously subjected to 3–5 firings between 800 and 850 °C for 2–3 days for each firing, except for Ba 0.78 Na 0.22 Fe 2 As 2 , which underwent two firings as above, and then was heated for 16 h at 1,000 °C for each of the last two anneals. Between each anneal, the powders were homogenized by grinding in a mortar and pestle. Annealing steps were kept as short as possible, enough to get chemically homogeneous powders while minimizing sodium loss, which is unavoidable. Before the last anneal, a slight amount of NaAs was added to compensate for the loss. The structure and quality of the final black powders were confirmed by x-ray powder diffraction and magnetization measurements. The magnetization curves of the measured samples are shown in Supplementary Fig. 1 . Powder diffraction The powder diffraction measurements were performed using two beam lines at the ISIS Pulsed Neutron Source, Rutherford Appleton Laboratory, UK: the high-resolution powder diffractometer, HRPD, and the cold-neutron powder diffractometer, Wish. The high resolution available at HRPD was necessary to resolve the weak orthorhombic splitting, while the high flux of Wish was required to measure the weak magnetic reflections. The same samples were used on both diffractometers within a few days of measurement. The results are summarized in the diffractograms (plots of intensity versus d -spacing and temperature), shown in Fig. 1 , with additional details provided by Supplementary Fig. 2 . How to cite this article: Avci, S. et al. Magnetically driven suppression of nematic order in an iron-based superconductor. Nat. Commun. 5:3845 doi: 10.1038/ncomms4845 (2014).